Dynamic scaling of morphogen gradients on growing domains Developmental mechanisms are highly conserved, yet act in embryos of very different sizes. How scaling is achieved has remained elusive. Here we identify a generally applicable mechanism for dynamic scaling on growing domains and show that it quantitatively agrees with data from the Drosophila wing imaginal disc. We show that for the measured parameter ranges, the Dpp gradient does not reach steady state during Drosophila wing development. We further show that both, pre-steady-state dynamics and advection of cell-bound ligand in a growing tissue can, in principle, enable scaling, even for non-uniform tissue growth. For the parameter values that have been established for the Dpp morphogen in the Drosophila wing imaginal disc, we show that scaling is mainly a result of the pre-steady-state dynamics. Pre-steady-state dynamics are pervasive in morphogen-controlled systems, thus making this a probable general mechanism for dynamic scaling of morphogen gradients in growing developmental systems. Spatial patterning during embryogenesis is controlled by morphogens that control tissue growth and differentiation at a distance from the cells that secrete them [1] . How morphogens are transported has remained controversial [2] , [3] , [4] . The proposed morphogen dispersal models can be divided into two categories: cell-based and diffusive [4] . Cell-based transport requires the endocytosis of ligand, and dynamin has indeed been shown to be important for morphogen spreading [5] . Internalized ligand can then be transported either by transcytosis [5] , a process by which macromolecules are transported across the interior of a cell, or by cytonemes, that is, by specialized filopodia that mediate long-distance signalling during development [6] , [7] . Diffusion of morphogens, either freely or hindered [3] , is well documented, but the relative contributions of the different transport mechanisms have remained controversial. According to the French Flag model [8] , cells read out the local morphogen concentration and respond when specific concentration thresholds are exceeded ( Fig. 1a ). To control patterning in embryos of different sizes with the same morphogen-based mechanism, the absolute positions where the threshold concentrations are reached need to shift between differently sized embryos ( Fig. 1b ). Different models have been proposed to explain the scaling of morphogen gradients in the various systems where scaling has been analysed [9] , [10] , [11] , [12] , [13] , [14] , [15] , [16] , [17] . However, these models have remained controversial because of conflicting experimental observations [16] , [18] , [19] , [20] , [21] . 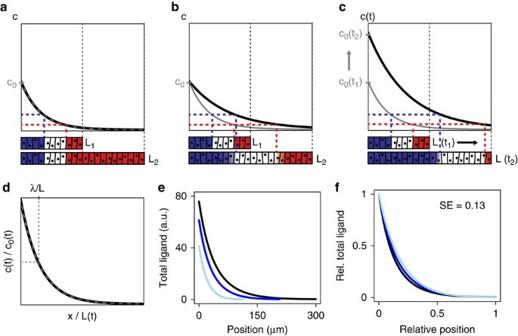Figure 1: Dynamic scaling of morphogen gradients on growing domains. (a) According to the French Flag model, concentration thresholds determine differential cell fate (blue, white and red) in a tissue. (b) To maintain proportions in differently sized tissue, gradients need to lengthen on longer domains. (c) Both the height,c0, and the length of the measured15Dpp gradient (equation (1)) increase on the growing wing imaginal disc of lengthL(t). (d) The measured15normalized Dpp gradients,c(t)/c0, of lengthλ(t)overlay on a rescaled domain,x/L(t). (e) The spreading of a morphogen gradient on a growing domain as a result of diffusion, advection and dilution in the absence of any reactions. Morphogens enter the domain at the left-hand side according to a flux boundary condition. The boundary at the right-hand side is impermeable, that is, we have zero-flux boundary conditions. For details, see Methods. (f) The normalized simulated gradient profiles fromeoverlay on the rescaled domain, that is, the gradients scale with domain size (cyan line: 24 h, blue line: 57 h, black line: 90 h). SE refers to the scaling error (equation 2) between the gradients att=24 h andt=90 h (0: perfect scaling; 1: no scaling; for details, see Methods). In all panels, the horizontal axis reports the position on the domain and the vertical axis reports concentration, as indicated. Figure 1: Dynamic scaling of morphogen gradients on growing domains. ( a ) According to the French Flag model, concentration thresholds determine differential cell fate (blue, white and red) in a tissue. ( b ) To maintain proportions in differently sized tissue, gradients need to lengthen on longer domains. ( c ) Both the height, c 0 , and the length of the measured [15] Dpp gradient (equation (1)) increase on the growing wing imaginal disc of length L(t) . ( d ) The measured [15] normalized Dpp gradients, c(t)/c 0 , of length λ(t) overlay on a rescaled domain, x / L(t) . ( e ) The spreading of a morphogen gradient on a growing domain as a result of diffusion, advection and dilution in the absence of any reactions. Morphogens enter the domain at the left-hand side according to a flux boundary condition. The boundary at the right-hand side is impermeable, that is, we have zero-flux boundary conditions. For details, see Methods. ( f ) The normalized simulated gradient profiles from e overlay on the rescaled domain, that is, the gradients scale with domain size (cyan line: 24 h, blue line: 57 h, black line: 90 h). SE refers to the scaling error (equation 2) between the gradients at t =24 h and t =90 h (0: perfect scaling; 1: no scaling; for details, see Methods). In all panels, the horizontal axis reports the position on the domain and the vertical axis reports concentration, as indicated. Full size image One such theory proposes that the production rate of the morphogen could be adjusted such that morphogen gradients are higher on larger tissues and thus keep a constant threshold concentration at the particular relative domain position, where the developmental pattern of interest is defined [16] . This model, however, does not apply to the Decapentaplegic (Dpp) gradient in the Drosophila wing and haltere imaginal discs, because measurements show that the gradients indeed widen with the expanding domain [15] . In parallel, however, also the maximal value of the gradients increases in the Drosophila wing and haltere imaginal discs, as well as in the early Drosophila embryo [9] , [14] , [15] , [22] ( Fig. 1c ), such that the measured gradients fall on the same curve (that is, scale) only when rescaled both relative to their maximal value and relative to the length of the domain ( Fig. 1d ). Accordingly, the Dpp concentration appears to increase with time for every single cell [15] ( Fig. 1c ). Absolute concentration measurements would then be insufficient to define a cell’s relative position in the domain. Interestingly, it has been reported that the concentration gradient of the downstream target of Dpp signalling, phosphorylated Mad, does not increase to the same extent as the Dpp gradient increases [23] . There may thus be an adaptation mechanism in place, which maintains stable response levels in spite of increasing absolute levels of Dpp ligand. Morphogen gradients can, in principle, also scale with domain size as a result of an appropriate adjustment of the diffusion and/or decay constants. These adjustments could be achieved either by passive or active modulators [16] . An active modulation mechanism for the Dpp gradient in the wing imaginal disc has recently been proposed [17] as an extension of a previously proposed expander–repressor scheme [13] . However, as recently noted, for this expander–repressor mechanism, the amplitude of the morphogen–receptor complex decreases more than twofold for a twofold increase in length, indicating that this mechanism is mainly based on an effective increase in the Dpp diffusion coefficient [16] . However, measurements in a range of systems, including the Drosophila wing imaginal disc, show that the (effective) diffusion coefficient of the ligand does not change, even though its gradient scales [15] . Scaling has therefore been suggested to be achieved by a reduction in the decay constant of the ligand on larger domains [15] ; the decay constant has not yet been directly measured on the expanding domain and experimental evidence for this proposal is therefore outstanding—as is a mechanism to achieve this reduction. It has recently been proposed that an expander–repressor mechanism based on an expander that reduces the Dpp decay rate could explain gradient scaling in the wing disc if the cellular growth rate was controlled by a relative change in Dpp signalling [24] . However, this previously proposed mechanism for growth control [15] has remained controversial, because clones in the wing imaginal disc that cannot transmit Dpp signalling grow at the same rate as signalling competent cells [25] . Moreover, the model fails to recapitulate the experimentally observed linear expansion of the wing disc domain with time [15] , but rather results in very fast initial growth and barely any domain expansion after about 50 h. As a result of the particular growth kinetics, advection and dilution contribute only to the early phases of growth in this model. Here we describe a general applicable mechanism for scaling of morphogen gradients on growing domains that recapitulates the quantitative measurements of the Dpp gradient in the Drosophila wing imaginal discs [15] , [23] , [26] . We show that both, pre-steady-state dynamics and advection of cell-linked ligand, can, in principle, result in scaling. For the parameter values that have been established for the Dpp morphogen in the Drosophila wing imaginal disc, scaling is, however, mainly the result of the pre-steady-state dynamics. The proposed mechanism also resolves the controversy related to Dpp transport in that it combines diffusion-based transport with cell-linked transport. The mechanism works for any ligand–receptor system if gradients are read out during a pre-steady state on a more or less uniformly growing tissue. Pre-steady-state dynamics and uniform growth are pervasive in morphogen-controlled systems, making it likely to be that the here-identified mechanism is of general use for scaled position-dependent readout in growing developmental systems. A measure of scaling We speak of scaling whether two gradients on differently sized domains overlay when normalized with respect to their maximal value and plotted on domains that have been normalized with respect to their maximal length, L . Accordingly, we can evaluate the quality of scaling by determining the scaling error (SE), , where Δ X specifies the difference of the normalized position X , at which a given normalized ligand concentration is attained by different gradients (for details see Methods). According to experimental data [15] , the Dpp gradients in the Drosophila wing imaginal disc remain of exponential shape as the disc is growing out, but the gradient lengthens such that the characteristic length λ increases with time t . The concentration gradients can therefore be well approximated by [15] where x denotes the position in the domain, with 0≤ x ≤ L(t) and x(t) = L(t)·X . We have perfect scaling between time points t 1 and t 2 , if . To obtain a measure of the SE, which is zero for perfect scaling and one for no scaling, we write For details on the derivation and calculation of SE, see Methods. Scaling by pre-steady state kinetics and advection To illustrate the mechanism of scaling, we first consider a very simple model of morphogen dynamics on a one-dimensional (1D) domain: Morphogens are produced on the left-hand side of the domain and enter the domain according to a flux boundary condition; we use an impermeable boundary on the other side (zero-flux boundary condition). Morphogens spread by diffusion; no reactions are included. The equations are given in the Methods. When we solve such a simple model on a growing domain, we find that the morphogen gradient expands over time ( Fig. 1e ) in a way that the gradient scales with domain size ( Fig. 1f ). Our model differs from previous studies of gradient scaling in that the simulated gradients do not reach their steady state within the physiological time scale, and in that the model is solved on a growing domain, such that we include advection and dilution. Dilution is an inevitable consequence of growth, that is, in the absence of any other processes the concentration of a component must decline as the domain expands because the number of molecules is fixed while the compartment size increases. Advection is inevitable if the ligand is attached to the moving domain, that is, if ligand is attached on cells or resides inside cells. In the Drosophila wing imaginal disc, at least 97% of all ligand has been found either internalized (>85%) or absorbed on cells, and <3% of all Dpp ligand is free in the extracellular space [26] , [27] , [28] . Cell-bound and internalized ligand cannot but move passively with the cells as the cells are pushed out during tissue growth ( Fig. 2a ). We illustrate this effect with a stable linear gradient of a compound, which is advected with the expanding domain in the absence of any diffusion or reactions ( Fig. 2b ). The gradient stretches with the expanding domain and the maximum of the gradient decreases due to dilution on the larger domain ( Fig. 2b , lighter grey lines). However, when rescaled with respect to the maximum concentration and the domain size, all lines perfectly overlay, that is, the gradients scale ( Fig. 2c ). The same holds true for an exponential gradient ( Fig. 2d,e ). For advection to be an efficient and functional transport mechanism, a large fraction of the ligand must be either bound to the cell surface or must be found inside cells [26] , [27] , [28] , internalized ligand–receptor complexes must remain stable for a long time, must be partitioned about equally during cell divisions [29] and must remain active after cell divisions [29] . All these conditions have previously been shown to apply to Dpp transport in the Drosophila wing imaginal disc [21] , [23] , [24] , [29] and are likely to also apply to other morphogen transport systems. 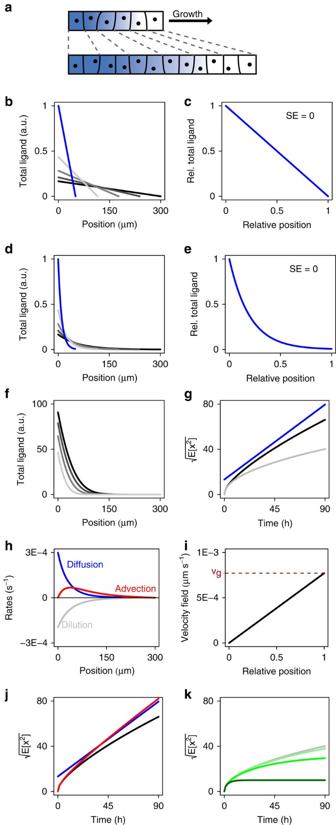Figure 2: Dynamic scaling as a result of pre-steady-state dynamics and advection. (a) As a result of advection, ligand on and inside cells is transported passively as cells are pushed out during tissue growth. (b) A stable non-diffusive linear gradient that experiences advection and dilution during growth expands on a growing domain (blue: initial gradient; light grey to black: increasing time steps). (c) The normalized gradients inbscale perfectly on the rescaled domain (SE=0, equation 2). (d,e) Perfect scaling (SE=0) does not depend on the shape of the stable gradient and also works for an initial exponential distribution. (f) The model shown inFig. 1e,fyields an expanding gradient also on a static, non-growing domain (length 300 μm), due to the pre-steady state (light grey to black: increasing time steps). (g) The mean-square displacement,E[x2], over time for the model that only includes advection and dilution (blue line, seeFig. 2dfor gradient profiles), for the model incorporating advection, dilution and diffusion (black line, seeFig. 1e,ffor gradient profiles), and for the model on the static, non-growing domain only incorporating diffusion (grey line, seeFig. 2ffor gradient profiles). The mean-square displacement of the diffusion-only model (grey line) perfectly follows the expectedcurve, while the advection-only model (blue line) expands linearly in time,~t(see Methods for a derivation); the model that includes both diffusion and growth lies in between those extremes (black line). (h) The relative contributions of the diffusion (blue), advection (red) and dilution (grey) terms on the temporal evolution of the total morphogen profile. (i) The velocity field on the scaled, uniformly growing domain. (j) Removal of the dilution term (red line) from the full model shown inFig. 1e,f, (black line) results in a more linearly increasing, similar as in the advection-only model (shown inFig. 1c) (blue line). (k) Higher degradation rates (increasing rates light to dark green) limit the expansion of the gradient compared with the purely diffusive model (grey line), and the gradients reach their steady-state profiles faster. For further details seeSupplementary Note 1. Figure 2: Dynamic scaling as a result of pre-steady-state dynamics and advection. ( a ) As a result of advection, ligand on and inside cells is transported passively as cells are pushed out during tissue growth. ( b ) A stable non-diffusive linear gradient that experiences advection and dilution during growth expands on a growing domain (blue: initial gradient; light grey to black: increasing time steps). ( c ) The normalized gradients in b scale perfectly on the rescaled domain (SE=0, equation 2). ( d , e ) Perfect scaling (SE=0) does not depend on the shape of the stable gradient and also works for an initial exponential distribution. ( f ) The model shown in Fig. 1e,f yields an expanding gradient also on a static, non-growing domain (length 300 μm), due to the pre-steady state (light grey to black: increasing time steps). ( g ) The mean-square displacement, E[x 2 ], over time for the model that only includes advection and dilution (blue line, see Fig. 2d for gradient profiles), for the model incorporating advection, dilution and diffusion (black line, see Fig. 1e,f for gradient profiles), and for the model on the static, non-growing domain only incorporating diffusion (grey line, see Fig. 2f for gradient profiles). The mean-square displacement of the diffusion-only model (grey line) perfectly follows the expected curve, while the advection-only model (blue line) expands linearly in time, ~ t (see Methods for a derivation); the model that includes both diffusion and growth lies in between those extremes (black line). ( h ) The relative contributions of the diffusion (blue), advection (red) and dilution (grey) terms on the temporal evolution of the total morphogen profile. ( i ) The velocity field on the scaled, uniformly growing domain. ( j ) Removal of the dilution term (red line) from the full model shown in Fig. 1e,f , (black line) results in a more linearly increasing , similar as in the advection-only model (shown in Fig. 1c ) (blue line). ( k ) Higher degradation rates (increasing rates light to dark green) limit the expansion of the gradient compared with the purely diffusive model (grey line), and the gradients reach their steady-state profiles faster. For further details see Supplementary Note 1 . Full size image Spreading of morphogens by diffusion is effective, however, also in the absence of growth ( Fig. 2f ), although the expansion is narrower ( Fig. 2g , grey line) than in the presence of growth ( Fig. 2g , black line). When we quantify the relative contributions of advection ( Fig. 2h , red line, Supplementary Fig. 1 ), dilution ( Fig. 2h , grey line), and diffusion ( Fig. 2h , blue line, Supplementary Fig. 1 ), we notice that transport by diffusion and dilution effects dominate close to the source, while advective transport dominates further away where the velocity field of the uniformly growing tissue is highest ( Fig. 2i ); we note that the velocity field on the rescaled, uniformly growing domain is constant over time. Importantly, although morphogen spreading as a result of advection is proportional to time ( Fig. 2g , blue line), diffusion-based spreading of ligand results in the expansion of the gradient proportional to the square root of time ( Fig. 2g , grey line); for details on the analysis, see Methods. In summary, only in case of advective transport, the gradient and the domain expand perfectly in parallel such that we have perfect scaling ( Fig. 2c,e ). The expansion of the gradients in Fig. 1e,f represents a mixture of these effects ( Fig. 2g , black line). In particular, we note that without dilution, the expansion of the gradients in Fig. 1e,f at later time points would be rather linear with time, as characteristic for transport by advection ( Fig. 2j , red line). On the other hand, incorporation of ligand degradation would severely limit the expansion of the morphogen gradient, and would result in a rapid formation of the steady-state profile ( Fig. 2k , green profiles). Dynamic scaling of the Dpp gradient in the wing disc In the Drosophila wing imaginal disc, most rate constants that relate to Dpp transport and signalling have been measured. This allows us to check the proposed scaling mechanism quantitatively with experimental data and to explore the relevance of the physiological values for the scaling mechanism. 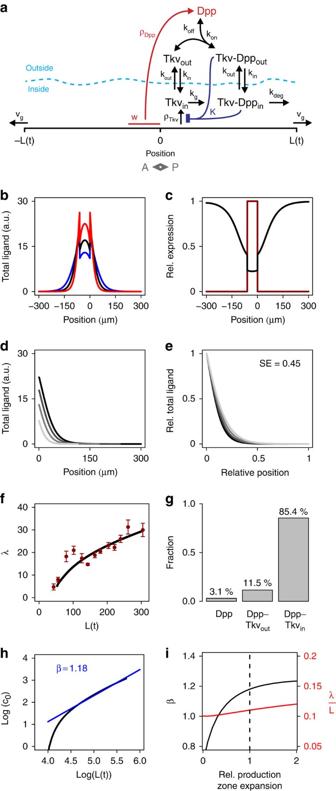Figure 3: The scaling mechanism reproduces the Dpp gradient characteristics from theDrosophilawing imaginal disc quantitatively. (a) The simulated Dpp network for theDrosophilawing imaginal disc. For details, see main text and Methods. (b) The parameters that affect the amount of receptor that is present outside affect the length of the gradient. Increasing the receptor production by twofold results in higher but shorter gradients (red), while decreasing receptor production by twofold results in wider but lower gradients (blue), as observed in experiments32. The black line shows the standard gradient. (c) The simulated expression profile of the Tkv receptor (black line) and of the Dpp ligand (red line). (d,e) The simulated gradient profiles of total Dpp (d) expand with the growing domain in a way that (e) the rescaled gradient profiles overlay on the rescaled domain. SE refers to the scaling error (equation (2)) between the gradients att=24 h andt=90 h. Time points shown (light to dark grey): 24, 46, 68, 90 h. (f) The length of the exponential gradient,λ(t), is about linearly related to the length of the domain,L(t), and matches the measured values (red)15. (g) The fraction of ligand that is unbound, bound to receptors on the membrane, or to internalized receptors matches the measured values15. The fractions were calculated based on the total concentration of each species in the whole posterior compartment. (h) With the exception of very early stages, the maximal value of the gradient,, and the length of the domain,L(t), are related according to a powerlaw,c0(t)=L(t)β(black line); the blue line shows the fitted line withβ=1.18; the linear fit was carried out between 10 and 90 h. (i) The exponentβof the power law depends on the relative speed, with which the ligand production zone and the target domain expand, and the measuredβis reproduced as long as the two domains expand together as observed in the experiment15. The relative expansion of the ligand-producing domain only has a very small effect on the length of the gradient,λ/L, and scaling is still observed if the ligand-producing domain does not expand. Figure 3a shows the Dpp signalling network. Dpp is produced at rate ρ Dpp in a narrow stripe at the boundary of the anterior (A) and posterior (P) compartments in the Drosophila wing imaginal disc, and the ligands diffuse into the target domain where they interact with their receptors (Tkv) on cells. Experiments demonstrate that most ligand is found inside cells [26] , [27] , [28] , and we therefore use a model [2] that also considers receptor binding and unbinding (at rates k on and k off ), and ligand internalization, and thus comprises diffusible ligand, internal and membrane-bound receptors, as well as receptor–ligand complexes ( Fig. 3a , Methods). The membrane-bound receptor–ligand complexes, Dpp-Tkv out , can be internalized ( k in ) and the internalized receptor–ligand complexes, Dpp-Tkv in , are either degraded ( k deg ) or exocytosed ( k out ) back to the membrane. Tkv receptors are produced throughout the domain ( ρ Tkv ). We extend the previous model [2] to also include a negative feedback of Dpp signalling via phosphorylated Mad on Dpp receptor (Tkv) production [30] , as well as a repressive effect close to the AP boundary due to Engrailed and Hedgehog signalling [31] , because experiments demonstrate that the receptor density affects both the height and the width of the gradient [32] , something that we also see in our simulations ( Fig. 3b ). The wild-type simulations reproduce the measured gradient in tkv expression and Tkv protein abundance, which are both lowest close to the dpp -expressing stripe [31] ( Fig. 3c and Supplementary Fig. 2 ).We solve the model on a growing 1D domain of length L(t) that spans the entire A–P axis of the Drosophila wing imaginal disc, that is, − L(t) ≤ x ≤ L(t) , with zero-flux boundary conditions at the ends of the domains. We note that given its simplicity, the model is sufficiently general to be applicable also to morphogens other than Dpp. The proliferation rate in the wing imaginal disc decreases over time inversely proportional to the area such that the domain expands linearly in size [15] . When we solve the model on a domain that expands linearly at the measured [15] growth speed v g , that is, L(t) = L(0)+v g t , we find that the resulting ligand gradient scales with the size of the patterning domain for physiological parameter values ( Supplementary Table 1 ). Thus, as the domain expands, both the maximal value and the reach of the ligand gradient increase ( Fig. 3d ), and the rescaled gradients overlay well ( Fig. 3e ). The scaling of the gradients is not perfect (according to equation 2, SE=0.45 between the gradients at 24 and 90 h). In spite of imperfect scaling, we note that the extent to which the gradients overlay is very similar to what is observed in experiments [15] in that the model has the same scaling properties as the Dpp gradient in the Drosophila wing disc. Thus, the simulations match the measured length of the Dpp gradient, λ(t) , versus the length of the wing disc domain, L(t) , over developmental time ( Fig. 3f ). The model also matches the measured distribution of ligand in unbound, internalized and surface-bound form ( Fig. 3g ). Thus, much as in measurements [26] , [27] , [28] , only about 3% of ligand represents free, extracellular ligand, while at least 85% of Dpp ligand resides inside cells and another 12% is absorbed on cells. Importantly, scaling is observed for all distinct ligand pools, that is, for the extracellular Dpp ligand alone ( Supplementary Fig. 3a ) and for the ligand–receptor complex, both if located on the extracellular membrane, Dpp-Tkv out ( Supplementary Fig. 3b ), or taken up by the cells, Dpp-Tkv in ( Supplementary Fig. 3c ). The signalling gradients thus also scale. The model also captures the increase of the maximal ligand concentration with domain size. Here the maximal ligand concentration is calculated as the sum of the Dpp, Dpp-Tkv out and Dpp-Tkv in concentration at the A–P compartment boundary ( x =0) and corresponds to c 0 in equation 1. Much as in the wing disc [15] , c 0 (t) and domain size are related according to a power law with exponent β =1.18 ( Fig. 3h ), which is twice the measured experimental value because the model is solved in one spatial dimension. The measured expansion of the Dpp-producing domain, the source, is necessary to recapitulate this aspect ( Fig. 3i , black line). Gradient scaling is, however, still possible also without any expansion of the source, both in simulations ( Fig. 3i , red line) and in mutants [15] . If the Dpp-producing tissue stripe cannot expand, the Dpp gradient is shorter, both in measurements [15] and simulations ( Fig. 3i , red line), because ligand production is reduced; a shorter gradient is also observed when reducing the ligand production rate ( Fig. 4a ) and the opposite behaviour is observed for the receptor production rate ( Fig. 4b ). Similarly, a higher receptor decay rate ( Fig. 4c ) and a higher ligand–receptor on-rate result in shorter gradients ( Fig. 4d ), while a higher ligand–receptor off-rate results in longer gradients ( Fig. 4e ). We note that these parameter values also affect the extent to which ligand is free, absorbed or internalized ( Fig. 4 , third column), but barely have an impact on the quality of scaling ( Fig. 4 , fourth and fifth columns) as judged by the SE. Here we note that the lower SE for higher ligand production rates ( Fig. 4a ) is the result of receptor saturation, and thus limited ligand turnover and higher effective diffusion; without receptor saturation, the ligand production rate would barely affect the scaling quality. To compare the quality of scaling by the eye, we rescaled the domains not only with respect to the length of the domain but also adjusted it with respect to the relative mean square displacement of the ligand (denoted Relative Normalized Position in Fig. 4 ); otherwise, the same relative SE would look worse for a wider gradient. Figure 3: The scaling mechanism reproduces the Dpp gradient characteristics from the Drosophila wing imaginal disc quantitatively. ( a ) The simulated Dpp network for the Drosophila wing imaginal disc. For details, see main text and Methods. ( b ) The parameters that affect the amount of receptor that is present outside affect the length of the gradient. Increasing the receptor production by twofold results in higher but shorter gradients (red), while decreasing receptor production by twofold results in wider but lower gradients (blue), as observed in experiments [32] . The black line shows the standard gradient. ( c ) The simulated expression profile of the Tkv receptor (black line) and of the Dpp ligand (red line). ( d , e ) The simulated gradient profiles of total Dpp (d) expand with the growing domain in a way that ( e ) the rescaled gradient profiles overlay on the rescaled domain. SE refers to the scaling error (equation (2)) between the gradients at t =24 h and t =90 h. Time points shown (light to dark grey): 24, 46, 68, 90 h. ( f ) The length of the exponential gradient, λ(t) , is about linearly related to the length of the domain, L(t) , and matches the measured values (red) [15] . ( g ) The fraction of ligand that is unbound, bound to receptors on the membrane, or to internalized receptors matches the measured values [15] . The fractions were calculated based on the total concentration of each species in the whole posterior compartment. ( h ) With the exception of very early stages, the maximal value of the gradient, , and the length of the domain, L(t) , are related according to a powerlaw, c 0 (t) = L(t) β (black line); the blue line shows the fitted line with β =1.18; the linear fit was carried out between 10 and 90 h. ( i ) The exponent β of the power law depends on the relative speed, with which the ligand production zone and the target domain expand, and the measured β is reproduced as long as the two domains expand together as observed in the experiment [15] . The relative expansion of the ligand-producing domain only has a very small effect on the length of the gradient, λ/L , and scaling is still observed if the ligand-producing domain does not expand. 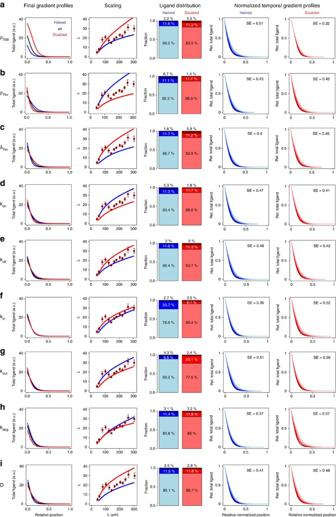Figure 4: The sensitivity and robustness of the scaling mechanism to changes in the parameter values. Influence of either doubling (red) or halving (blue) the specified model parameters of the full model shown inFig. 3(as given inSupplementary Table 1), that is, of the (a) Dpp production rate, (b) Tkv production rate, (c) Tkv degradation rate, (d) Dpp-Tkv binding rate, (e) Dpp-Tkv unbinding rate, (f) Tkv internalization rate, (g) Tkv exocytosis rate, (h) degradation rate of internalized Dpp, (i) Dpp diffusion constant, on the gradient shape at 90 h (first column), on gradient scaling (second column) and on the fractions of the different Dpp ligand populations (Dpp-Tkvin: light shading; Dpp-Tkvout: intermediate shading; Dpp: dark shading) (third column). Influence of either halving (fourth column) or doubling (fifth column) the specified model parameters of the full model shown inFig. 3(as given inSupplementary Table 1) on scaling of the normalized gradients on the rescaled domain. Some parameter values affect the spread of the gradient, but not the scaling. To correct for the effects of different positions on the gradient profiles, we normalized the domain with the relative change in the gradient dispersal, that is, Relative Normalized Position=[Absolute Position/L(t)] ·. SE refers to the scaling error (equation (2)) between the gradients att=24 h andt=90 h (0: perfect scaling; 1: no scaling; for details, see Methods). Full size image Figure 4: The sensitivity and robustness of the scaling mechanism to changes in the parameter values. Influence of either doubling (red) or halving (blue) the specified model parameters of the full model shown in Fig. 3 (as given in Supplementary Table 1 ), that is, of the ( a ) Dpp production rate, ( b ) Tkv production rate, ( c ) Tkv degradation rate, ( d ) Dpp-Tkv binding rate, ( e ) Dpp-Tkv unbinding rate, ( f ) Tkv internalization rate, ( g ) Tkv exocytosis rate, ( h ) degradation rate of internalized Dpp, ( i ) Dpp diffusion constant, on the gradient shape at 90 h (first column), on gradient scaling (second column) and on the fractions of the different Dpp ligand populations (Dpp-Tkv in : light shading; Dpp-Tkv out : intermediate shading; Dpp: dark shading) (third column). Influence of either halving (fourth column) or doubling (fifth column) the specified model parameters of the full model shown in Fig. 3 (as given in Supplementary Table 1 ) on scaling of the normalized gradients on the rescaled domain. Some parameter values affect the spread of the gradient, but not the scaling. To correct for the effects of different positions on the gradient profiles, we normalized the domain with the relative change in the gradient dispersal, that is, Relative Normalized Position=[Absolute Position/ L(t) ] · . SE refers to the scaling error (equation (2)) between the gradients at t =24 h and t =90 h (0: perfect scaling; 1: no scaling; for details, see Methods). Full size image The quality of scaling mainly depends on the pre-steady-state dynamics of the gradient and is therefore highest for slow ligand turnover, that is, for low rates of receptor internalization, k in ( Fig. 4f ), for high rates of receptor exocytosis, k out ( Fig. 4g ), and for a low degradation rate, k deg ( Fig. 4h ). The internalization rate of the BMP and TGF-β receptors has been measured in several cell culture systems and half the receptor is internalized within 5–15 min, both in the presence and absence of ligand [33] , [34] , [35] , corresponding to a rather high effective internalization rate of 0.8–2.3 × 10 −3 s −1 . We use the most conservative value of k in =0.8 × 10 −3 s −1 in the model; we note that twofold deviations from this value barely affect the scaling properties of the system, but have an impact on the fraction of extracellular and internalized ligand ( Fig. 4f ). The receptor-related rates and the binding rates also affect the fraction of extracellular ligand and the gradient length ( Fig. 4b–e ). We set these rates to typical physiological values ( Supplementary Table 1 ) that allow us to reproduce the measured fractions. We note that the different rates compensate for each other ( Fig. 4 ), such that there is a wide range of parameter sets that allows us to match the experimental measurements. As degradation rate of internalized ligand, we use k deg =4 × 10 −6 s −1 , which corresponds to a half-life of internalized Dpp of 48 h. The low degradation rate of internalized ligand ensures that gradient formation is slow ( Fig. 2k ), such that the gradient does not reach steady state during wing disc development, as required for the scaling mechanism. The long half-life of internalized ligand is in apparent contradiction to the fast clearance of Dpp ligand in the experiments by Teleman and Cohen [28] . However, in those experiments only very little intracellular Dpp was detected, and the measured clearance rate thus mainly represented the loss of extracellular ligand, as also noted in the previous analysis by Lander et al. [2] Given the fast rate of ligand internalization, this aspect is also captured by our model. The Dpp degradation rate that was reported by Gonzalez-Gaitan and colleagues [15] , [26] , on the other hand, was inferred from the measured length of the Dpp gradient and the Dpp diffusion coefficient, but was not measured. Thus, the reported reduction in the Dpp degradation rate over time [15] does not represent an actual experimental observation but only reflects the predicted behaviour of the Dpp degradation rate for the case that scaling was obtained with a steady-state Dpp gradient. As our model reproduces the Dpp gradient length with the diffusion coefficient measured by Gonzalez-Gaitan’s team, our simulation is also in agreement with these data. Here we note that measurements of the Dpp diffusion constant range between 0.1 (refs 15 , 26 ) and 20 μm 2 s −1 (ref. 27 ). Even though small changes in the diffusion coefficient already affect the gradient shape ( Fig. 4i ), a higher diffusion coefficient can be compensated by a higher receptor–ligand affinity ( Fig. 4d,e ) and/or higher receptor abundance ( Fig. 4b,c,f,g ) to arrive at the same measured gradient length ( Fig. 5a ); in that case, however, there is considerably less free extracellular ligand. As the exact fraction of extracellular ligand is difficult to establish experimentally, the entire range of measured diffusion coefficients is, in principle, consistent with the proposed gradient scaling mechanism. Similarly, we note that with a fivefold higher degradation rate, which corresponds to a half-life of internalized Dpp of <10 h, we still obtain scaling and we still match the measured Dpp gradient length, λ(t) , versus the length of the wing disc domain, L(t) , over developmental time ( Fig. 5b ). A half-life of at least 10 h is supported by previous observations, according to which internalized Dpp ligand remains active beyond cell divisions [29] ; the cell cycle time is 6–30 h in wing imaginal discs [15] . Our proposed scaling mechanism is therefore consistent with all these previous measurements. 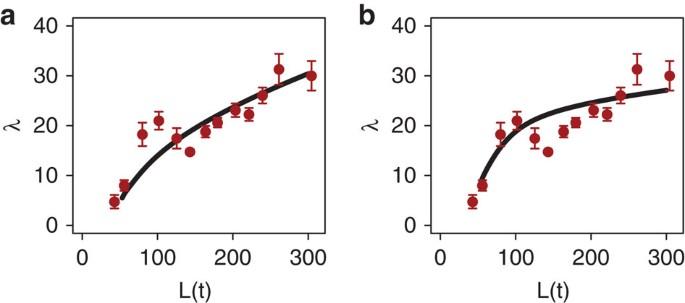Figure 5: Alternative model parameterizations quantitatively fit the experimental data. The predicted length of the exponential gradient,λ(t), at different domain lengths,L(t), (solid line) and the measured values (red dots)15. (a) A 100-fold higher diffusion coefficient can be compensated by a 100-fold higher Dpp-Tkv binding rate (kon). However, the predicted fraction of free ligand would then be much smaller than 1%. (b) A fivefold higher degradation rate (kdeg=2 × 10−5s−1) can be compensated by a slightly higher diffusion coefficient (DDpp) and a slightly higher Dpp-Tkv binding rate (kon). All quantitative data, including the fraction of free ligand, would still be reproduced. The alternative parameterizations are listed inSupplementary Table 1. Figure 5: Alternative model parameterizations quantitatively fit the experimental data. The predicted length of the exponential gradient, λ(t) , at different domain lengths, L(t) , (solid line) and the measured values (red dots) [15] . ( a ) A 100-fold higher diffusion coefficient can be compensated by a 100-fold higher Dpp-Tkv binding rate ( k on ). However, the predicted fraction of free ligand would then be much smaller than 1%. ( b ) A fivefold higher degradation rate ( k deg =2 × 10 −5 s −1 ) can be compensated by a slightly higher diffusion coefficient ( D Dpp ) and a slightly higher Dpp-Tkv binding rate ( k on ). All quantitative data, including the fraction of free ligand, would still be reproduced. The alternative parameterizations are listed in Supplementary Table 1 . Full size image How uniform does growth need to be for gradients to scale Finally, we wondered to what extent gradient scaling would depend on uniform growth. When we either restrict all growth to a small part of the domain ( Fig. 6a ) or set growth to zero in a small part of the domain ( Fig. 6b ), as is the case in certain clones, gradient scaling is barely affected as long as the overall growth of the whole domain is linear. Scaling can thus be still obtained in case of non-uniform linear growth. Scaling is even observed if the domain grows only at the tip ( Fig. 6c ). In that case, there is no advective transport, and indeed, when we quantify the contributions of diffusion, advection and dilution in the wing disc model ( Fig. 3a ) we find that transport by diffusion dominates close to the source ( Fig. 6d and Supplementary Fig. 1 ), even though only 3% of ligand is free ( Fig. 3g ). In line with this, the experimentally established gradient length, λ(t) , versus the domain length, L(t) , can be fitted by a square root function ( Fig. 6e ) as characteristic for a purely diffusive, pre-steady-state transport process ( Fig. 2g , Methods). We note, however, that there are limits to the extent to which non-uniform growth can be tolerated: for exponentially growing domains, the SE increases considerably (SE=0.53 for the exponentially growing domain versus SE=0.45 for the linearly growing domain) ( Fig. 6f ). The fact that the SE is still so small can be accounted to the impact of advection, which is considerably stronger on an exponentially growing domain ( Supplementary Fig. 4 ). For comparison, increasing k deg fivefold while leaving all other parameter values unchanged (such that the steady state is attained much more quickly) results in SE=0.82 on a linearly growing domain. 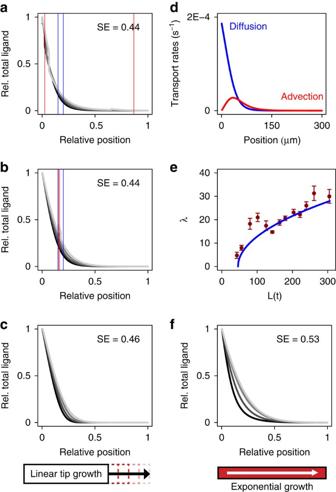Figure 6: Relative contributions of diffusion and advection on ligand transport in theDrosophilawing disc model. (a) A small clone that solely contributes to the observed growth (no growth outside the clone) has only minor impact on gradient scaling as long as the total domain size grows linearly. Blue vertical lines indicate the initial boundaries of the clone; red vertical lines indicate the boundaries of the clone in the final domain. (b) A small non-growing clone does not influence scaling as long as the total domain size grows linearly. Blue vertical lines indicate the initial boundaries of the clone; red vertical lines indicate the boundaries of the clone in the final domain. (c) Linear tip growth (no advection) only slightly affects the quality of scaling. (a–c) SE refers to the scaling error (equation (2)) between the gradients att=24 h andt=90 h (0: perfect scaling; 1: no scaling; for details, see Methods). (d) The influence of advection of the bound (and therefore advected) ligand species is very small compared with the diffusion of the free ligand, suggesting that the influence of advection is negligible in the wing disc and scaling is mainly obtained by a diffusion-based pre-steady-state expansion of the gradient. The calculation was carried out at the final time point,t=90 h. (e) The measured length of the exponential gradient,λ(t), at different lengths,L(t), of the wing disc (red dots)15can be fitted with a square-root function of domain length (which itself is linearly related to time), thus supporting a diffusion-based pre-steady-state gradient expansion (for details, see Methods). (f) Gradients do not scale on an exponentially growing domain. SE refers to the scaling error (equation (2)) between the gradient att=40 h andt=90 h (0: perfect scaling; 1: no scaling; for details, see Methods). Note that the exponentially growing domain at 40 h has the same length as the linearly growing domain at 24 h. For further details, seeSupplementary Note 2. Figure 6: Relative contributions of diffusion and advection on ligand transport in the Drosophila wing disc model. ( a ) A small clone that solely contributes to the observed growth (no growth outside the clone) has only minor impact on gradient scaling as long as the total domain size grows linearly. Blue vertical lines indicate the initial boundaries of the clone; red vertical lines indicate the boundaries of the clone in the final domain. ( b ) A small non-growing clone does not influence scaling as long as the total domain size grows linearly. Blue vertical lines indicate the initial boundaries of the clone; red vertical lines indicate the boundaries of the clone in the final domain. ( c ) Linear tip growth (no advection) only slightly affects the quality of scaling. ( a – c ) SE refers to the scaling error (equation (2)) between the gradients at t =24 h and t =90 h (0: perfect scaling; 1: no scaling; for details, see Methods). ( d ) The influence of advection of the bound (and therefore advected) ligand species is very small compared with the diffusion of the free ligand, suggesting that the influence of advection is negligible in the wing disc and scaling is mainly obtained by a diffusion-based pre-steady-state expansion of the gradient. The calculation was carried out at the final time point, t =90 h. ( e ) The measured length of the exponential gradient, λ(t) , at different lengths, L(t) , of the wing disc (red dots) [15] can be fitted with a square-root function of domain length (which itself is linearly related to time), thus supporting a diffusion-based pre-steady-state gradient expansion (for details, see Methods). ( f ) Gradients do not scale on an exponentially growing domain. SE refers to the scaling error (equation (2)) between the gradient at t =40 h and t =90 h (0: perfect scaling; 1: no scaling; for details, see Methods). Note that the exponentially growing domain at 40 h has the same length as the linearly growing domain at 24 h. For further details, see Supplementary Note 2 . Full size image Conclusion In summary, the simulations establish that scaling of the Dpp morphogen gradient on the linearly, uniformly growing wing disc domain is the result of the pre-steady-state dynamics of the ligand ( Figs 3 , 4 , 5 , 6 ). The large amount of available quantitative experimental data allowed us to quantitatively test the proposed mechanism: the model recapitulates the measurements in the Drosophila wing disc quantitatively, and resolves the controversy related to Dpp transport and readout in that it combines diffusion-based transport with cell-linked transport. Further experiments will nonetheless be of interest. In particular, it will be important to confirm the rather long half-life of internalized Dpp ligand explicitly, which ensures that the gradient dynamics are in pre-steady state. According to our analysis, the half-life should be at least 10 h, but much longer half-lives (~48 h) are likely. In contrast to a recently proposed model for morphogen gradient scaling [24] , it is not necessary that the morphogen controls growth to achieve scaling. Gradient scaling and domain growth can therefore be independently controlled processes that are linked via advection. Ligand transport by advection, in principle, enables perfect scaling on a uniformly expanding domain ( Fig. 2b–e ), because the gradient then expands in parallel with the expanding domain (see Methods for details), as required for scaling. However, transport by advection has only little effect on gradient scaling in the wing disc relative to diffusion ( Fig. 6 ), because the growth field of the uniformly growing domain is rather small close to the ligand source ( Fig. 2i ), and because dilution and degradation of internalized ligand limit the quality of scaling ( Fig. 2j,k ). There is a general requirement for gradient scaling during embryogenesis as well as during the evolution of differently sized species. Pre-steady-state dynamics and (quasi-) uniform, linear growth are pervasive in morphogen-controlled systems, making it probable that the here-identified mechanism is of general use for scaled position-dependent readout in growing developmental systems. A simple model for ligand dynamics on a growing domain In the simple models, for which we show results in Figs 1e,f and 2 , we only consider a ligand with concentration c(x,t) , which diffuses with diffusion coefficient D =0.005 μm 2 s −1 on a growing 1D domain, x ε[0, L ( t )] with L(t)=L(0)+v g t , where t denotes time. We note that the diffusion constant had to be chosen much smaller than the measured range ( D =0.1 μm 2 s −1 (refs 15 , 26 ) to D =20 μm 2 s −1 (ref. 27 )), because in this simple model we do not include any reactions that would limit the length of the gradient to its physiological length. Over the 90 h of development, the wing disc domain expands from an initial size L(0) =50 μm to a final size of L(90 h) =300 μm [15] . The measured growth speed is thus with L(t) = L(0)+v g t . Based on Reynolds transport theorem, the diffusion equation for c on a growing domain is given by Here, u denotes the growth field, is the advection term, is the dilution term and is the diffusion term. Reactions are not included in this simple model. Dilution is a natural consequence of growth. The inclusion of the advection term is justified only if the ligand is transported by the growing tissue. This is the case if most functional ligand is bound on cells or is inside cells, as has indeed been reported for Dpp in the Drosophila wing imaginal disc [26] , [27] . To model the influx of ligand from the producing domain, we use flux-boundary conditions with flux j in =10 −14 μm −1 on the left-hand side ( x=0 ). The boundary condition on the right-hand side ( x=L(t) ) has little impact on the model, because the ligand concentration on the right-hand side is rather low; we chose zero-flux boundary conditions, that is, As initial conditions we are using c(x,0) =0. The growth field u for a uniformly growing domain is given by A model for the Dpp gradient in the Drosophila wing disc We base our model on a previously published model for Dpp ligand dynamics in the Drosophila wing imaginal disc [2] . The model considers both the diffusible ligand Dpp and the cell-bound receptor Tkv . Ligands can bind to receptors at the cell surface at rate k on to form the Dpp-Tkv complex Dpp-Tkv out , and unbind at rate k off . The receptor–ligand complex is not degraded on the cell surface, but is rather internalized at rate k in ; the internalized Dpp-Tkv complex, Dpp-Tkv in , can still signal. The internalized complex, Dpp-Tkv in , is then either degraded at rate k deg or transported back to the membrane at rate k out . Dpp production is restricted to a small domain just anterior to the boundary of the A and P compartments. The measurements of the Dpp gradient are typically carried out in the posterior compartment, and we will therefore solve the model on a 1D domain centred at the A–P boundary, which itself is posterior to the Dpp-expressing cells. The ligand-producing domain is denoted by Λ Dpp and the expression rate of Dpp by ρ Dpp . The receptor, Tkv , is produced inside cells at rate ρ Tkv throughout the target domain and reaches the cell surface by exocytosis. Accordingly, we include an internal and an external receptor species in the model, denoted by Tkv in and Tkv out , respectively. The unbound and bound receptors appear to be endocytosed at similar rates [33] . As these measurements are of limited precision, we use identical rates in the model. Thus, the internal Tkv receptor, Tkv in , is exocytosed at rate k out and unbound, external receptor, Tkv out , is endocytosed at rate k in . As an extension to the previously published model [2] , we now include the well-described details of the regulation of tkv expression in the model as well, because the resulting spatially modulated receptor profiles can affect the spatial ligand dynamics [32] . The expression of tkv in Drosophila is downregulated both by Dpp and Hh signalling [30] , [31] . We include the downregulation by Dpp signalling via an inhibiting Hill term that depends on the concentration of bound Dpp-Tkv receptor, that is, Hh signalling induces the expression of dpp and reduces the expression of tkv . We do not include Hh dynamics in the model explicitly, but rather decrease ρ Tkv by twofold in the Dpp-producing domain Λ Dpp . ρ Tkv (x) is therefore defined as: In summary, the reaction terms R i for the components c i in Fig. 3a in the main paper are given as Unlike in the previous publication of the model [2] , we solve the model on a growing domain and thus formulate the model as advection-reaction-diffusion equations for a compound c i with diffusion coefficient D i , velocity field u and reaction terms R i : According to experimental data, the wing disc is expanding linearly with time, and we therefore solve the model on a linearly growing 1D domain, x ε[− L ( t ), L ( t )] with According to measurements, the ligand-producing stripe expands as the wing disc is growing, that is, The receptors are restricted to cells and their diffusion coefficient is therefore set to zero. We use zero flux boundary conditions for all components, that is, The absolute protein concentrations in the wing imaginal disc have not been established. We therefore use non-dimensionalized protein concentrations. It is likely to be that receptor is initially distributed uniformly, and accordingly we use an initially spatially uniform, non-dimensional concentration for the receptor concentration on the surface, Tkv out . The initial internal receptor concentration, Tkv in is set to the ratio of the production and degradation rates, that is, . For the free ligand and for both internal and external receptor–ligand complexes, we use zero as initial conditions, that is, Parameter values The parameter values that are used in our standard model are listed in Supplementary Table 1 . Based on experiments, the initial size of the wing disc was set to L(0) =50 μm and the developmental time was set to 90 h [15] . The final imaginal disc size is about 300 μm (ref. 15 ), and accordingly the growth rate was set to . The internalization rate was set according to measurements. Thus, measurements in a wide range of systems show that half of the Dpp ligand is internalized within 10–15 min [33] , [34] , [35] , that is, k in =0.8–2.3˙10 −3 s −1 ; we use a conservative internalization rate, that is, k in =0.8˙10 −3 s −1 . The exocytosis rate has not yet been established. We use k out =1˙10 −4 s −1 to obtain the measured fraction of internalized ligand, ≥85% (refs 2 , 27 ). Two important parameter values in the model that deserve further discussion are the diffusion coefficient, D , and the degradation rate, k deg . Measurements by different groups have resulted in very different values for the Dpp diffusion constant, with reported values ranging between 0.1 (refs [15] , [26] 15,26) and 20 μm 2 s −1 (ref. 27 ). As shown in Figs 3d–f and 5a , scaled gradients can be obtained over the entire measured range, because the diffusion coefficient can be compensated by adjusting the ligand–receptor binding affinity ( k on , k off ) and/or the receptor abundance in the model, that is, ρ Tkv , k out , k in or δ Tkv , all of which have not yet been measured. Accordingly, the entire range of measured diffusion coefficients is consistent with currently available experimental data. However, it has to be noted that for a given gradient width, there is only one diffusion coefficient that yields the measured fraction of free ligand, because the diffusion coefficient is the only parameter for which the gradient width and the fraction of free ligand change in opposite directions as the parameter value is changed ( Fig. 4i ). The affinities and the receptor expression/degradation rates, on the other hand, regulate the width of the gradient and the fraction of free ligand in the same direction ( Fig. 4b–e ). We used the Dpp diffusion coefficient, D Dpp =0.1 μm 2 s −1 , which was reported in the Kicheva et al. [26] publication, because it resulted in the measured fraction of free ligand of 3% (refs 26 , 27 ); the other above mentioned parameter values that have an impact on the gradient length and fraction of free ligand were adapted accordingly. We stress here that although D Dpp =0.1 μm 2 s −1 was uniquely best suited to reproduce the reported distribution of ligand, the measurements of the ligand fractions are too imprecise as that they would exclude different diffusion coefficients. Moreover, there are a number of processes that affect the effective diffusion that we do not include in the model (for example, binding to the extracellular matrix). The second important parameter value is k deg , which determines the time scale on which the gradient reaches its steady-state profile. This rate has so far not been determined explicitly, and the many indirect measurements are unsuitable to infer its value as discussed in the main text. We use k deg =4˙10 −6 s −1 as turnover rate for internalized Dpp, which corresponds to a half-life of internalized Dpp of 48 h. We note that scaling and a similar fraction of internalized Dpp can still be obtained with a fivefold higher turnover rate ( k deg =2˙10 −5 s −1 ) for internalized Dpp ( Fig. 5b ). Previous estimates had suggested k deg ≥10 −4 s −1 , but these were based on a steady-state assumption [2] , [15] , [26] . A steady-state assumption implies a high degradation rate such that the ‘prediction’ of a high degradation rate directly follows from the specific assumption of a steady-state gradient; we now show that such a steady-state assumption does not hold with physiological parameters. For more details, see the Results section. In summary, we set all parameter values to be within the probable physiological range ( Supplementary Table 1 ), but we note that a wide range of parameter sets would be consistent with the available data; the exact values are thus not identifiable, but also do not matter for the analysis of the scaling mechanism. Gradient expansion in the simple ligand model In Fig. 2 we analysed how diffusion, advection and dilution affect the expansion of the gradient, c , in the simple model, that is, . To quantify the dispersion of c(x,t) , we determined the mean squared displacement As before, L(t) = L(0)+v g t denotes the domain length. As expected, we observed that for advection increases linearly with respect to time, while in case of diffusion increases with the square root of time. In particular, we found that for an exponential initial profile with characteristic length λ , , and for the diffusion-only transport . Here we derive these relationships. Influence of diffusion on gradient expansion In Fig. 2d we solved equations (1, 2, 3) on a static domain. On a static domain, there are no advection and dilution effects, and transport is thus purely a result of diffusion. We therefore deal with the simple 1D diffusion equation For a Dirac delta function δ ( x ) as an initial condition, the solution to the diffusion equation on an infinite domain is which is the normal distribution with mean μ =0 and variance σ 2 =2 Dt . The variance σ 2 =2 Dt is twice the value obtained in our simulations, E [ x 2 ]= Dt . This difference can be accounted to the flux-boundary condition in our model. Thus, although the right-hand boundary has little effect as long as the domain is sufficiently large, the ligand source at the left-hand boundary prevents us from using an infinite domain approximation. Rather, we need to consider the diffusion equation on a semi-infinite domain ( x ε[0,∞]). If we use f(x) as initial condition and homogeneous Neumann boundary conditions in the first instance, we obtain Using again the Dirac Delta function as initial condition, that is, f(x) = δ(x) , and the property of the Delta function , this simplifies to which is the half-normal distribution with σ 2 =2 Dt . The variance is the second central moment of a random variable U, that is, Var ( U )= E [ U 2 ]−( E [ U ]) 2 . Therefore, we can write E [ U 2 ]= Var ( U )+( E [ U ]) 2 and, given the variance and mean of the half-normal distribution, we have . This is the same expectation value of x 2 as in the normal distribution. In our model, we still have a slightly different situation in that we have a constant influx at the left-hand side boundary instead of a given initial distribution. We can approximate our inhomogeneous Neumann boundary condition at x =0 as a mixture distribution of half-normal distributions with different end times t end , where and i =0,1,2, ... , k . For large k , the following is therefore a good approximation E [ x 2 ] of this mixed distribution is then the weighted sum of the individual expectation values, , which range from E i=0 [ x 2 ]=0 to E i=k [ x 2 ]=2 Dt . As E i ∝ t , we have as observed in our simulations of the simple ligand-only model on a static domain ( Fig. 2g , grey line). In summary, in case of diffusion, increases with the square root of time. Influence of advection on gradient expansion Now we consider ligand transport on a uniformly growing domain L(t) = L(0)+v g t in the absence of diffusion. Transport by advection (in the absence of diffusion) applies if all ligands are strictly attached or within a cell and the domain is growing. We then have Given that we have linear, uniform growth, we have and dilution is thus spatially uniform, such that the gradient height decreases uniformly, while the gradient shape remains preserved. Assuming that we have some initial distribution U with initial mean μ 0 =0 and initial variance σ 0 =0, we can again write . To analyse the impact of growth, we consider a scaled distribution V(t) such that . We now use that Var ( aU )= a 2 Var ( U ) and E [ aU ]= aE [ U ], such that E [ V 2 ]= a 2 ( Var ( U )+( E [ U ]) 2 ). With , we thus have . We now consider a concentration profile on an infinite domain z ε[0,∞]. We then have E [ z 2 ]=2 λ 2 . To capture the impact of growth from L(0) to L(t) , we use the mapping , and have as indeed observed in the simulations. In summary, in case of advection, increases linearly with the linearly expanding domain, and thus linearly with time. Contribution of diffusion and advection to ligand transport Both, in the simple model as given by equation (3) and in the detailed model for the Dpp gradient in the Drosophila wing imaginal disc as given by equations (8, 9), diffusion and advection contribute to ligand transport. Supplementary Fig. 1 quantifies the relative contributions of the two transport modes. In both models, transport by diffusion dominates close to the source ( Supplementary Fig. 1a,e,i, m ), while transport by advection dominates far away from the source ( Supplementary Fig. 1c,g,k,o ), because transport by advection is still strong, while transport by diffusion is negligible; there is no transport by advection on the right-hand-side boundary. Transport by advection is strongest slightly away from the source ( Supplementary Fig. 1b,f,j,n ), where the velocity field u is of intermediate strength ( Fig. 2i ), while the gradient of the ligand concentration is still high ( Supplementary Fig. 1d,h,l,p ). Far away from the source, >90% of all Dpp transport can be accounted to advection ( Supplementary Fig. 1k )—even though no more than 80% of Dpp in the outer parts got there by advection ( Supplementary Fig. 1o ). In the simple model, transport rates by diffusion and advection both decline over time ( Supplementary Fig. 1a,b ). On the other hand, in the more detailed model, transport rates by diffusion and advection both increase over time ( Supplementary Fig. 1i,j ). This can be accounted to the different descriptions of ligand production. In the simple model, we use a flux boundary condition on the left-hand-side boundary, while in the detailed wing disc model, ligand is produced continuously in the expanding stripe in the centre of the domain. As a result, the spatial ligand gradient at the left-hand-side declines at later times in the simple model, but continues to increase in the more detailed model, thereby supporting increased transport by both diffusion and advection. Evaluation of scaling quality We speak of scaling if two gradients on differently sized domains overlay when normalized with respect to their maximal value and plotted on domains that have been normalized with respect to their maximal length. To evaluate the quality of scaling, we seek to determine the extent, to which the gradients are shifted over time on the normalized domain, X ε[0,1]. Accordingly, we define the SE as , where Δ X specifies the difference of the position X at which a given normalized concentration is attained by the different gradients. According to experimental data, the Dpp gradients in the Drosophila wing imaginal disc remain of exponential shape as the disc is growing out, but the gradient lengthens such that the characteristic length of the gradient, λ , increases [15] . We therefore now consider exponential gradients of the form with x(t) = L(t)X , and L(t) is the size of the domain at time t . We have perfect scaling if To evaluate the SE between two gradients at two different time points t 1 and t 2 , we consider the two normalized gradients and on the rescaled domain . We then have , which yields , and thus . The SE is then We note that this corresponds to determining in the λ(t) versus L(t) plot in Fig. 3f as a measure of scaling. As expected, the SE is zero if and approaches one in the limit L ( t )→∞ as t →∞ if λ (t) =const., i.e., if the gradient does not lengthen on a growing domain. For a finite time t 2 , the maximal SE is obtained with λ(t 2 )= λ(t 1 ) such that . To obtain a measure for the SE, which is zero for perfect scaling and one for no scaling, we use To calculate the SE for the gradients in our models we need to determine their characteristic length λ(t) at different time points. In principle, this could be done by fitting an exponential function to the simulation results and determining the characteristic length from the fit. However, such fittings are imprecise, and we rather use that E [ z ]= λ for an exponential gradient on z ε[0,∞]. Accordingly, we can approximate α in equation (25) by calculating E[X] for two normalized, rescaled gradients at two different time points t 1 and t 2 , that is, As expected, if the two gradients are identical and thus α =1, the SE is zero. Moreover for t →∞, we have L ( t 2 )→∞ and thus α →0, SE →1. For a finite time t 2 , the maximal SE is now . Software The equations were solved with finite difference methods as implemented in MATLAB on uniform growing domains, and by finite element methods as implemented in COMSOL Multiphysics 4.3b on non-uniformly growing domains [36] , [37] . How to cite this article: Fried, P. et al. Dynamic scaling of morphogen gradients on growing domains. Nat. Commun. 5:5077 doi: 10.1038/ncomms6077 (2014).